8.4% efficient fullerene-free organic solar cells exploiting long-range exciton energy transfer In order to increase the power conversion efficiency of organic solar cells, their absorption spectrum should be broadened while maintaining efficient exciton harvesting. This requires the use of multiple complementary absorbers, usually incorporated in tandem cells or in cascaded exciton-dissociating heterojunctions. Here we present a simple three-layer architecture comprising two non-fullerene acceptors and a donor, in which an energy-relay cascade enables an efficient two-step exciton dissociation process. Excitons generated in the remote wide-bandgap acceptor are transferred by long-range Förster energy transfer to the smaller-bandgap acceptor, and subsequently dissociate at the donor interface. The photocurrent originates from all three complementary absorbing materials, resulting in a quantum efficiency above 75% between 400 and 720 nm. With an open-circuit voltage close to 1 V, this leads to a remarkable power conversion efficiency of 8.4%. These results confirm that multilayer cascade structures are a promising alternative to conventional donor-fullerene organic solar cells. Organic solar cells are a potential low-cost alternative to conventional inorganic solar cells due to their ease of processing and compatibility with flexible substrates [1] , [2] . The power conversion efficiency (PCE) of organic photovoltaic (OPV) devices has increased rapidly in the last decade [3] , partly owing to adaptations of the device architecture. Following the introduction of the donor/acceptor (DA) interface by Tang [4] , the bulk heterojunction [5] , [6] and the tandem structure [7] , [8] have been the most explored device architectures to increase PCE. Further efficiency enhancements have primarily been related to the development of improved donor materials [9] , [10] . On the other hand, fullerene molecules and their derivatives have become the dominant acceptor materials in OPV cells due to their good electron-accepting ability and high electron mobility [11] , [12] . However, the small absorption overlap with the solar spectrum limits the photocurrent generation in fullerene acceptors. Furthermore, the relatively small electrical bandgap of the fullerene acceptor can limit the open-circuit voltage ( V OC ) in these devices [13] . These shortcomings have stimulated the development of non-fullerene acceptors in recent years [14] , [15] . Alternatives to fullerenes for vacuum-deposited small-molecule organic solar cells mainly comprise perylene derivatives [4] or halogenated (sub-)phthalocyanines [16] , [17] , [18] . However, these non-fullerene acceptors rarely show improved performance over their fullerene counterparts. To illustrate, the best non-fullerene-based OPV cell reported up to now, consisting of a boron subphthalocyanine chloride (SubPc) donor and a fused fluorinated SubPc dimer acceptor, achieves a PCE of 4% (ref. 17 ), which is comparable to the best bilayer SubPc/C 60 cells reported in the literature [19] . Additionally, it has been shown that non-halogenated SubPc, mostly known as a donor material, can act as an electron-accepting material in bilayer OPV cells [20] . Using a tetracene donor layer to supply the required energy level offset at the DA heterojunction, a PCE of 3.1% can be obtained [21] despite the low electron mobility and low electron affinity of SubPc used as acceptor [22] . The main performance improvement in this case stems from the ability to achieve significantly higher V OC compared with the fullerene acceptor. This is due to the higher lowest unoccupied molecular orbital (LUMO) level of SubPc. The use of non-fullerene acceptors thus provides a way to improve energy level alignment of the DA heterojunction and simultaneously enhance light absorption by better overlap with the solar spectrum. Another approach to increase the photocurrent generation in organic solar cells is the incorporation of additional light-absorbing materials besides the required donor and acceptor, as in ternary blend bulk heterojunction devices [23] , [24] , [25] . In planar heterojunction devices, several mechanisms have been proposed to extract photocurrent from an additional active layer. In a three-layer stack with cascade-energy-level-alignment, a centered ambipolar layer can enable double exciton dissociation at both interfaces with the donor and acceptor, increasing the photocurrent generation in the cell [21] , [26] . However, this is at the expense of the voltage generated by the solar cell, as the V OC is ultimately limited by the energy levels of the outer layers in such a cascade structure. Alternatively, in an energy-relay cascade structure, excitons in a large-bandgap donor material are transferred by interlayer exciton energy transfer to a smaller-bandgap donor, and subsequently dissociated at the interface with the acceptor [27] , [28] . In this device architecture, a broad part of the solar spectrum can be covered by combining materials with complementary optical properties, and, significantly, a decrease in V OC can be avoided by aligning the highest occupied molecular orbital (HOMO) energy levels of the multiple donor materials. However, previous reports have not fully exploited these advantages, and OPV devices with substantial efficiency enhancement have not yet been shown. Here, we present small-molecule organic solar cells with non-fullerene electron-accepting materials. We first show SubPc and its homologue boron subnaphthalocyanine chloride (SubNc) can act as acceptors in bilayer devices with an α-sexithiophene (α-6T) donor ( Fig. 1a ). With efficiencies up to 6%, these devices exceed the performance of fullerene-based devices. When both acceptors are combined in a three-layer device structure the photocurrent generation is further increased, with a two-step exciton-dissociating mechanism shown to be active ( Fig. 1b,c ). The resulting PCE of 8.4% is unprecedented for fullerene-free organic solar cells, and even establishes a record efficiency for evaporated single-junction OPV devices. 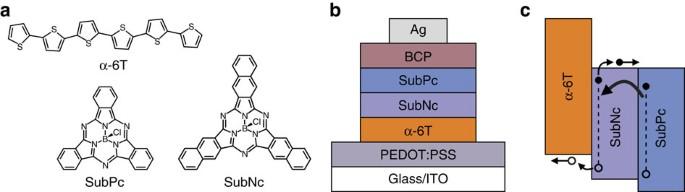Figure 1: Three-layer device architecture with interlayer energy transfer. (a) Molecular structures of the active materials. (b) Schematic representation of the device architecture. (c) Energy-level diagram of the active layers illustrating the two-step exciton dissociation mechanism. Figure 1: Three-layer device architecture with interlayer energy transfer. ( a ) Molecular structures of the active materials. ( b ) Schematic representation of the device architecture. ( c ) Energy-level diagram of the active layers illustrating the two-step exciton dissociation mechanism. Full size image Bilayer devices Bilayer heterojunction devices were fabricated on indium tin oxide-coated glass substrates with the following layer structure: poly(3,4-ethylenedioxythiophene):poly(styrenesulfonate) (PEDOT:PSS)/α-6T/ A /bathocuproine (BCP)/Ag, where the acceptor A is C 60 , SubPc or SubNc. Current density–voltage ( J-V ) characteristics of these devices were measured under simulated solar illumination of 100 mW cm −2 . The nominal thickness of the α-6T donor layer is fixed at 60 nm, considering it does not significantly influence the device performance within a certain thickness range [29] . The thickness of the acceptor layer and the BCP layer were optimized to maximize PCE for each device structure ( Table 1 ). We notice the optimal thickness of the BCP exciton-blocking layer is different for each acceptor material, as it has a large influence on the device performance [30] . Compared with the reference device with a C 60 acceptor, both V OC and short-circuit current density ( J SC ) are significantly improved for devices with SubPc or SubNc as acceptor ( Fig. 2 ), resulting in PCE values of 4.7% and 6.0%, respectively. Considering that previous efforts to use typical donor molecules as acceptor have not succeeded to exceed the efficiency of fullerene-based devices, these results present an important advance in the field of fullerene-free organic solar cells. Table 1 Performance characteristics for the reported device architectures. 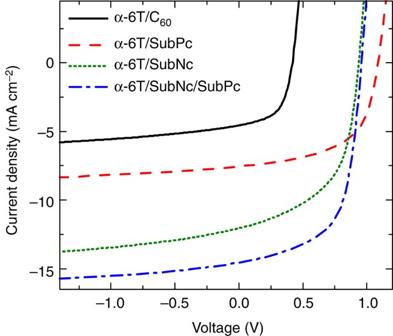Figure 2: Device performance of fullerene-free OPV devices. Compared with the acceptor C60, non-fullerene acceptors SubPc and SubNc increase theVOCandJSCof bilayer devices with an α-6T donor. The photocurrent generation is further increased by exploiting interlayer FRET in a three-layer device architecture. Full size table Figure 2: Device performance of fullerene-free OPV devices. Compared with the acceptor C 60 , non-fullerene acceptors SubPc and SubNc increase the V OC and J SC of bilayer devices with an α-6T donor. The photocurrent generation is further increased by exploiting interlayer FRET in a three-layer device architecture. Full size image The high photocurrent generation in the fullerene-free devices is in the first place attributed to the strong absorption by SubPc and SubNc in visible light. Both materials have an absorption coefficient of 3.5 × 10 5 cm −1 at their peak wavelength. Furthermore, the absorption spectra of these materials complement the α-6T donor ( Fig. 3a ), and both layers contribute to the photocurrent as evidenced by the measured external quantum efficiency (EQE) spectra ( Fig. 3b ). The internal quantum efficiency (IQE) was estimated by dividing the EQE spectrum by the absorption of each device (measured via reflection, including parasitic absorption, and thus serving as a lower bound for IQE). High IQE values of 70% for the SubPc acceptor and 85% for the SubNc acceptor are obtained. This is facilitated by the high surface roughness of the underlying α-6T donor layer. Atomic force microscopy images indicate an RMS roughness of 15.9 nm and a 37% increase in surface area compared with the projected area ( Supplementary Fig. 1 ). Most excitons generated in the acceptor layer can therefore reach the DA interface and dissociate, resulting in high IQE values. 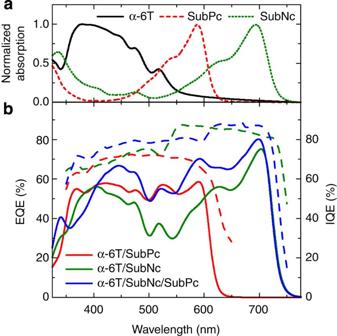Figure 3: Spectral response of fullerene-free OPV devices. (a) The absorption spectra of the three active materials complement each other to effectively harvest solar light. (b) The measured EQE (solid lines) and IQE (dashed lines) spectra show efficient photocurrent generation by all three absorbing materials. Figure 3: Spectral response of fullerene-free OPV devices. ( a ) The absorption spectra of the three active materials complement each other to effectively harvest solar light. ( b ) The measured EQE (solid lines) and IQE (dashed lines) spectra show efficient photocurrent generation by all three absorbing materials. Full size image The substantially higher V OC of the fullerene-free devices results from improved energy level alignment between the frontier molecular orbitals at the DA interface. The V OC of organic heterojunction devices is primarily determined by the interface gap, that is, the energy difference between the HOMO of the donor and the LUMO of the acceptor [31] . Both SubPc and SubNc have a LUMO energy level of −3.6 eV (refs 32 , 33 ), considering the extension of the conjugated system is mainly associated with a shift of the SubNc HOMO [34] , [35] . With the HOMO of α-6T around −5.0 eV (ref. 36 ), an interface gap of ~1.4 eV exists for the α-6T/SubPc and α-6T/SubNc heterojunctions. This results in a much lower energetic loss compared with the α-6T/C 60 heterojunction, which induces an interface gap of only 0.8 eV (ref. 29 ). The α-6T/SubNc device showed a strong decrease in FF when the thickness of the SubNc acceptor layer was increased, an aspect that can often be attributed to difficult extraction of the generated charges. Zero-field electron mobilities of 4.9 × 10 −6 and 4.2 × 10 −9 cm 2 V −1 s −1 were determined for SubPc and SubNc, respectively ( Supplementary Fig. 2 ). Despite the low electron mobility of the SubNc acceptor, no increase in series resistance was observed in dark J-V measurements of bilayer devices with thick SubNc layers. Therefore, we conclude the low FF in these devices is not related to a limited charge extraction through the acceptor layer. The decrease in FF is rather related to a voltage-dependent photocurrent in the fourth quadrant of the J-V curve. In the α-6T/SubPc device this effect is absent, and the FF does not significantly decrease for SubPc thicknesses below 20 nm. Three-layer device Similar to an energy-relay cascade structure with multiple donor materials, SubPc and SubNc can be combined as acceptors in a three-layer device structure. The SubNc layer, positioned in the middle of the three-layer stack, can function both as an electron acceptor and as an energy acceptor for excitons generated in α-6T and SubPc, respectively. Such a three-layer device structure was fabricated by sequentially depositing SubNc and SubPc on top of the α-6T donor layer ( Fig. 1b ). Again, the thickness of both acceptor layers and the BCP layer were adjusted to maximize the PCE ( Table 1 ). The thickness of the SubNc layer could be reduced with respect to the bilayer α-6T/SubNc device. The additional SubPc layer eliminates the need for a thick SubNc layer by altering the optical interference pattern in the organic layers, ensuring strong absorption even in a thin SubNc layer. Similar to the bilayer device, the reduced SubNc thickness results in a high FF. Furthermore, an increase in photocurrent generation is observed in the three-layer device structure, whereas the V OC structure is similar to the α-6T/SubNc device ( Fig. 2 ). As mentioned above, because SubNc and SubPc have similar LUMO energy levels, a decrease in V OC is circumvented, contrary to previously reported cascade structures [21] , [27] . This results in an improved performance for the three-layer energy cascade structure, with the best performing device generating a PCE of 8.4%, surpassing the current state-of-the-art evaporated single-junction OPV devices [37] , [38] . For certification purposes, devices with a 1-cm 2 active area were fabricated and measured in-house with an average PCE of 7.81%, and 7.93% for the best performing device. This device was certified at Newport Corporation PV Lab with a PCE of 7.77% (±0.16%) ( Supplementary Fig. 3 ). Compared with the bilayer α-6T/SubNc device, the EQE spectrum of the three-layer device shows an additional peak at 590 nm, corresponding to the absorption peak of SubPc ( Fig. 3b ). This confirms the additional SubPc layer is actively contributing to the photocurrent, and not merely acting as a transport layer aiding the extraction of electrons. The resulting IQE surpasses 75% in a broad wavelength range from 400 to 720 nm. Two mechanisms can explain the contribution by SubPc to the photocurrent. First, the SubNc/SubPc interface can function as a one-sided heterojunction where only excitons from the SubPc side are dissociated due to the HOMO energy level offset between SubPc and SubNc. This energy offset is estimated at only 0.2 eV, which is smaller than the exciton-binding energy of most organic semiconductors. As a consequence, the dissociation of SubPc excitons at this interface might be inefficient. Alternatively, a two-step exciton dissociation mechanism can explain the SubPc contribution to the photocurrent. This mechanism comprises Förster resonance energy transfer (FRET) from SubPc to SubNc, and consequent charge transfer at the α-6T/SubNc interface. Mediated by dipole–dipole interactions, FRET is a long-range exciton transfer process occurring between a luminescent energy donor and an absorptive energy acceptor [39] . The Förster transfer rate from an emissive donor molecule to a layer of acceptor molecules is given by Scully et al. [40] where ρ A is the molecular density of the energy acceptor, τ is the natural exciton lifetime in the emissive layer and d the distance between the emitting molecule and the quenching layer. The Förster radius of energy transfer R 0 depends on the spectral overlap between the emission of the energy donor and the absorption of the energy acceptor. To examine the significance of the interlayer FRET mechanism in our three-layer α-6T/SubNc/SubPc device, a set of photoluminescence (PL) quenching experiments was performed. Modeling the experimental results allows to extract the Förster radius R 0 , as demonstrated in the work of Luhman and Holmes [41] . A three-layer structure is used to spatially separate the energy donor from the energy acceptor. An inserted wide-bandgap spacer layer suppresses exciton quenching by direct charge transfer at the interface, whereas long-range energy transfer across the transparent spacer layer is still possible. The interlayer energy transfer efficiency is then evaluated from the PL quenching for different spacer thicknesses. The measured PL intensity is directly proportional to the exciton density n in the emissive donor layer. Simulated exciton density profiles are obtained by solving the steady-state one-dimensional exciton diffusion equation, modified to incorporate interlayer energy transfer: where D is the exciton diffusion coefficient, Q ( x ) is the exciton generation rate as calculated from a transfer matrix method, and k f is given by equation (1). Here, the molecular separation distance d will depend on the position x in the emissive layer. Numerical solutions of equation (2) are used to fit experimental PL data with R 0 as a fitting parameter. Here, quartz substrates were coated with a 20-nm-thick SubPc layer, a 4,4′-Bis( N -carbazolyl)-1,1′-biphenyl (CBP) spacer layer with varying thickness, and a 10-nm SubNc quenching layer. Samples with C 60 as quenching layer were used as control structures as negligible energy transfer is expected due to the limited absorption overlap of C 60 with SubPc emission. Emission spectra were measured both with and without quenching layers to determine the PL ratio for each CBP thickness ( Supplementary Fig. 4 ). The emission spectrum of SubPc consists of two distinct peaks centered at 620 and 710 nm (ref. 42 ). Because the peak at longer wavelengths partially overlaps with the emission of SubNc, the signal was deconvoluted and the PL intensity was obtained by integrating the deconvoluted SubPc signal between 685 and 745 nm ( Supplementary Fig. 5 ). We directly observe that SubNc quenches the SubPc PL signal substantially compared with a C 60 quenching layer ( Fig. 4 ). This indicates FRET from SubPc to SubNc is very efficient and long-range interlayer exciton transfer is possible. In fact, the PL signal is still effectively quenched by SubNc for spacer layers up to 35 nm. The experimental PL ratios were fitted using numerically simulated exciton density profiles from equation (2), where an exciton diffusion length of 6 nm was used for SubPc, as extracted from thickness-dependent PL quenching experiments ( Supplementary Fig. 6 ). The simulation results nicely fit the experimental PL ratios, considering the slight deviation at low spacer layer thickness is likely caused by an underestimation of the SubNc contribution to the measured PL signal. A value of 7.5 nm for R 0 was extracted for exciton energy transfer from SubPc to SubNc, whereas no significant energy transfer is observed with a C 60 quenching layer ( R 0 <1 nm). 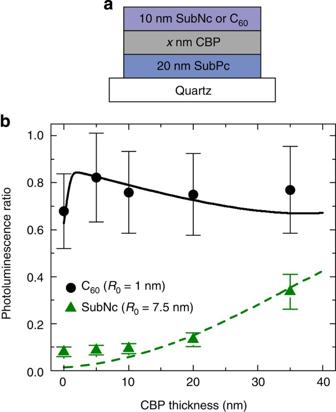Figure 4: Evaluation of exciton energy transfer efficiency. (a) Schematic representation of the layer structure used in PL quenching experiments. (b) Experimental PL ratios indicate effective quenching of the SubPc PL signal by energy transfer to the SubNc quenching layer. Numerical modeling of these results (solid lines) allows to extract the Förster radius of energy transferR0. Error bars for the PL ratio are determined from the root mean square difference between the experimental data and the analytical model resulting from the peak-fitting algorithm. Figure 4: Evaluation of exciton energy transfer efficiency. ( a ) Schematic representation of the layer structure used in PL quenching experiments. ( b ) Experimental PL ratios indicate effective quenching of the SubPc PL signal by energy transfer to the SubNc quenching layer. Numerical modeling of these results (solid lines) allows to extract the Förster radius of energy transfer R 0 . Error bars for the PL ratio are determined from the root mean square difference between the experimental data and the analytical model resulting from the peak-fitting algorithm. Full size image The high extracted Förster radius confirms the suggested two-step exciton dissociation mechanism in the three-layer α-6T/SubNc/SubPc device ( Fig. 1c ). Excitons generated in the SubPc acceptor layer are transferred to the intermediate SubNc layer, and subsequently diffuse toward the interface with the α-6T donor, where an exciton dissociation process occurs. Considering R 0 was extracted for organic layer stacks with planar interfaces, we expect the efficiency of the energy transfer process to be further enhanced in the three-layer device structure due to the high interface roughness induced by the underlying α-6T layer ( Supplementary Fig. 1 ). Because the underlying α-6T layer contains several tall grains, direct contact between SubPc and α-6T might occur due to incomplete coverage of these tall grains by the intermediate SubNc layer. This would result in an additional dissociation mechanism for SubPc excitons. Due to the short exciton diffusion length, however, only the excitons in a limited volume of the SubPc layer are prone to this charge generation pathway. Exciton diffusion in SubPc is most likely based on self-Förster energy transfer, with an estimated self-Förster radius of 1.5 nm (ref. 43 ). Considering the obtained Förster radius of 7.5 nm, excitons at the SubNc/SubPc heterojunction are transferred more efficiently to SubNc by interlayer FRET compared with diffusion toward possible α-6T/SubPc interfaces. The suggested two-step charge generation mechanism including energy transfer will therefore be dominant. The efficient exciton energy transfer from SubPc to SubNc is mainly a consequence of their complementary optical properties: there is a good spectral overlap between the emission of SubPc and the absorption of SubNc. In general, the Stokes shift of the energy donor should match the difference between the optical bandgap of the energy donor and the energy acceptor. However, this Stokes shift should not be too large, as this corresponds to the energy loss accompanying the interlayer energy transfer process. Besides these requirements, other material properties that determine the FRET efficiency were not considered for the material system reported in this work. For example, the molecular orientation in the amorphous SubPc and SubNc layers is assumed to be isotropic, and the transition dipole moments are not aligned for the energy transfer process. Therefore, control of the molecular orientation, for instance by introducing templating layers, could be considered in the search for alternative material systems with an efficient interlayer exciton energy transfer process. In summary, we have demonstrated that subphthalocyanines SubPc and SubNc can be used as electron acceptors in highly efficient organic solar cells. In discrete bilayer heterojunction devices with an α-6T donor and SubPc or SubNc as acceptor, we realize PCE values of 4.7 and 6%, respectively, both higher than previously reported values for fullerene-free devices. The combination of strong absorption in the non-fullerene acceptors and a large DA interface area results in high quantum efficiencies. In addition, high V OC values are realized in these fullerene-free OPV devices due to the enhanced energy level alignment between donor and acceptor. Exploiting long-range FRET, SubPc and SubNc can be combined as acceptors in a three-layer device structure, with a two-step exciton-dissociating mechanism shown to be active. Excitons generated in the outer SubPc acceptor are transferred to the middle SubNc layer and consequently dissociated at the remote α-6T/SubNc interface. The SubNc layer thus functions simultaneously as an energy acceptor for excitons generated in the SubPc layer, and as a charge acceptor at the interface with α-6T. The demonstrated PCE of 8.4% is extraordinarily high for a fullerene-free device, and even exceeds the performance of previously reported vacuum-deposited single-junction organic solar cells utilizing fullerenes. Due to long-range exciton harvesting by interlayer energy transfer, the multilayer energy cascade structure thus forms an important alternative to conventional device architectures for improving the performance of organic solar cells. Thin film and device preparation Organic thin films for PL quenching experiments were deposited on quartz substrates, and OPV devices were fabricated on pre-patterned indium tin oxide-coated glass substrates. Detergent and solvent cleaning of all substrates was followed by a 5 min oxygen–plasma treatment to remove the remaining carbon residue. Spin-coating of a 20 nm-thick layer PEDOT:PSS was followed by a bake-out at 130 °C in N 2 . All organic materials used in this study were purified by thermal gradient sublimation before loading in a high-vacuum evaporation chamber, where they were deposited at a rate of 1 Å s −1 . The 120-nm-thick Ag cathode was evaporated at 3 Å s −1 through a shadow mask, defining an active area of 13.4 mm 2 . Devices with a 1-cm 2 active area were encapsulated and wire-bonded for certification at the Newport Corporation PV Lab. Optoelectronic characterization Current density–voltage characteristics were measured under simulated solar illumination, using a Keithley 2602 measurement unit and an Abet solar simulator, calibrated with a Fraunhofer certified photovoltaic cell to yield a 100 mW cm −2 AM1.5G spectrum. For the EQE measurements, light from Xe and quartz halogen lamps was coupled into a monochromator and their intensities were calibrated with a Si photodiode. The light incident on the device was chopped and the modulated current signal was detected with a current–voltage and lock-in amplifier. The same optics and measurement set-up was used with a DTR6-integrating sphere to determine the reflection R . IQE values were determined as EQE/(100%− R ). Morphological characterization The topography of organic films deposited on Si/SiO 2 substrates was studied by atomic force microscopy using an Agilent 5100 scanning probe operated in tapping mode. Electron mobility measurements To determine the electron mobilities of SubPc and SubNc the J-V characteristics of electron-only devices were measured. These devices consisted of a 100 nm-thick organic layer inserted between two Yb-doped BCP layers as the electron-injecting contacts. The results were fitted to a space-charge-limited-current model described by , where ε 0 is the permittivity of free space, and the relative permittivity of the organic layer is assumed ε =4. The zero-field mobility μ 0 and the field activation parameter γ are used as fitting parameters, whereas V and L are the applied voltage and the thickness of the organic layer, respectively. PL intensity measurements PL quenching experiments were performed using a N 2 laser with pulse duration of 1.2 ns operated at 20 Hz for optical excitation at 532 nm. The samples were excited through the quartz substrate at an incidence angle of 45° to the substrate normal. Emission spectra were recorded using a triple-grating monochromator coupled to an intensified CCD camera (PI-MAX from Princeton Instruments), which was synchronized by the electrical trigger of the laser. To increase the signal-to-noise ratio, spectra were accumulated by averaging over 2,000 pulses. The reported PL ratios were calculated for the peak at 710 nm in the SubPc emission spectrum. As this peak partially overlaps with emission of SubNc, the signal was deconvoluted using a peak-fitting algorithm ( Supplementary Fig. 5 ). After subtraction of the background signal of the peak at lower wavelength, the measured PL signal was fitted with two Gaussian-shaped curves centered around the wavelength of maximum emission of SubPc and SubNc thin films, at 710 and 720 nm respectively. The PL intensity was obtained by integrating the fitted curve corresponding to SubPc emission between 685 and 745 nm. This method was used to analyze all organic layer stacks containing a SubNc quenching layer. For stacks without SubNc quenching layer (no quenching layer or a C 60 quenching layer), a single Gaussian curve was used to fit the experimental PL signal and calculate the integrated intensity. Exciton density simulations and fitting procedure Exciton density profiles were simulated by numerically solving the steady-state one-dimensional exciton diffusion equation modified to incorporate interlayer energy transfer (equation (2)). A value of 1.5 nm −3 was used for the molecular density of the energy acceptor ρ A . The exciton generation rate Q ( x ) was taken from the optical absorption profile calculated from a transfer matrix method, using optical constants measured by spectroscopic ellipsometry. The integrated exciton density profiles were assumed to be directly proportional to the PL intensity, and could therefore be used to fit the experimentally obtained PL ratios. This fitting was performed using a least mean squares fitting algorithm, using the exciton diffusion length and the Förster energy transfer radius R 0 as fitting parameters. Assuming energy transfer from SubPc to C 60 is negligible, the SubPc exciton diffusion length was first extracted from thickness-dependent PL quenching experiments, using a C 60 quenching layer ( Supplementary Fig. 6 ). A value of 6 nm was obtained. This value was subsequently used in simulations for organic layer stacks including a spacer layer, where R 0 was used as fitting parameter. The CBP spacer layer and the quartz substrate were both assumed to form non-quenching interfaces. How to cite this article: Cnops, K. et al. 8.4% efficient fullerene-free organic solar cells exploiting long-range exciton energy transfer. Nat. Commun. 5:3406 doi: 10.1038/ncomms4406 (2014).